Graphene radio frequency receiver integrated circuit Graphene has attracted much interest as a future channel material in radio frequency electronics because of its superior electrical properties. Fabrication of a graphene integrated circuit without significantly degrading transistor performance has proven to be challenging, posing one of the major bottlenecks to compete with existing technologies. Here we present a fabrication method fully preserving graphene transistor quality, demonstrated with the implementation of a high-performance three-stage graphene integrated circuit. The circuit operates as a radio frequency receiver performing signal amplification, filtering and downconversion mixing. All circuit components are integrated into 0.6 mm 2 area and fabricated on 200 mm silicon wafers, showing the unprecedented graphene circuit complexity and silicon complementary metal–oxide–semiconductor process compatibility. The demonstrated circuit performance allow us to use graphene integrated circuit to perform practical wireless communication functions, receiving and restoring digital text transmitted on a 4.3-GHz carrier signal. With recent developments in graphene field-effect transistors (GFETs) showing intrinsic unity current gain frequencies ( f T ) higher than 400 GHz (ref. 1 ), along with theoretical work projecting operation exceeding 500 GHz (ref. 2 ), graphene shows great promise in radio frequency (RF) applications. The rapid advances in graphene transistor performances, f T and maximum oscillation frequency ( f MAX ), came from all aspects of the device, including improved starting graphene materials [3] , better gate dielectrics [4] , [5] , [6] , improved contact resistance [7] , new device architectures [8] , [9] and aggressive channel length scaling [1] , [10] . On the other hand, the pace of the development of graphene RF circuits seems significantly slower, and raises the question about the true feasibility of using graphene in modern communication systems. Most graphene circuits demonstrated today are arguably the extension of the study of a transistor itself. High-performance discrete passive components have been connected to GFET externally at the equipment level, and these circuits are limited to single-transistor designs. Demonstrations using this approach have shown several promising GHz functions such as voltage amplification [11] , frequency multiplication [12] , [13] and signal mixing [7] , [14] . However, to compete with existing technologies, particularly silicon, requires that all active and passive components be monolithically integrated onto single chip for not only the small circuit footprint and low cost but also high circuit complexity and advanced system functionality. A millimetre-wave mixer integrating exfoliated graphene and microstrip technology has recently been demonstrated [15] . The circuit fabrication, however, requires more exotic processes such as substrate thinning and through-substrate via etching. For the large-scale synthesized graphene, perhaps the best attempt displayed to date is a single-stage mixer integrated circuit (IC) built by small-piece, offline-type processes [16] . This proof-of-concept IC consists of only one transistor, fabricated by a conventional process flow, that is, the active device was first constructed, followed by a series of back-end-of-line (BEOL) processes to complete the circuit interconnect and passive components. Because of the delicacy of graphene, resulting from its single atomic layer nature and weak adhesion between graphene and other materials, these BEOL processes inevitably deteriorate GFET quality, which is evident from much worse device performance in the IC compared with stand-alone GFETs using similar substrates [3] , [4] , [10] , [17] . This fundamental process compatibility issue apparently hinders the progress of graphene RF research. Here, we present the first multi-stage graphene RF IC fabricated in a standard silicon fab. The device integrity is fully preserved and the circuit performance is confirmed by the demonstration of successful receiving and recovering of digital text carried on a GHz signal. The device degradation issue is overcome by completely reversing the conventional fabrication flow, where all passive components together with device gates are first built on 8-inch silicon wafers before the graphene films, grown by chemical vapour deposition (CVD) methods [18] , are transferred. The demonstrated conversion gain at the same local oscillator (LO) input power is ~10,000 × better than previously reported graphene IC [16] . This novel integration scheme can also be applied to any channel materials that can be transferred, such as carbon nanotubes [19] or other two-dimensional nanomaterials [20] , [21] . 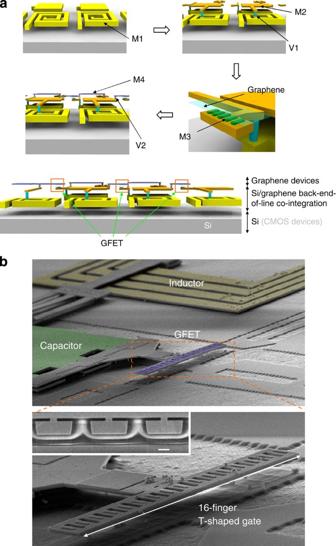Figure 1: Fabrication and architecture of graphene receiver IC. (a) Schematic of the passive-first active-last process flow showing how the IC fabrication can be integrated into standard Si BEOL process. Four metal levels (M1–M4) are required to complete the circuit. (b) Tilted view scanning electron microscopic (SEM) image revealing the integration of key components in IC with enlarged view showing the advanced gate structure of the graphene field-effect transistors (GFET). Inset image shows cross-sectional SEM of embedded T-shaped gate. Scale bar, 500 nm. Passive-first active-last fabrication flow Figure 1a shows schematics of the simplified fabrication flow, which depicts the establishment of the passive-first active-last integration scheme. Inductors and bottom plate of capacitors were first fabricated at M1 metal level using single Cu damascene process. To get high-quality factor ( Q ) of the inductors, M1 was thicker than 1 μm, and can be the same top metal level in standard Si complementary metal–oxide–semiconductor (CMOS) chips for global power distribution. The fabricated inductors showed inductances matching the designed values ( Supplementary Table 1 ) with Q >8 ( Supplementary Fig. 1 ). The M2 metal level formed by the similar Cu damascene process served as the top plate of capacitors as well as the bottom (wide) part of the embedded T-shaped gate. The M3 metal lines were then patterned to form the top part of the T-shaped gate, where the width of M3 lines defined the transistor’s channel length. After the T-gate formation, atomic layer deposition (ALD) was used to deposit gate dielectric of 10 nm Al 2 O 3 followed by CVD graphene transfer and patterning. The mobility of the CVD graphene is around 2,000–2,500 cm 2 (Vs) −1 at the carrier density of 2 × 10 12 cm −2 ( Supplementary Fig. 2 ). No seed layers that are typically needed for promoting the nucleation of gate dielectric on graphene were required, resulting in high gate dielectric quality and the potential for future scaling. As the last step, the M4 metal level comprising Pd/Au stack was deposited to form resistors and also device source/drain contacts. Figure 1: Fabrication and architecture of graphene receiver IC. ( a ) Schematic of the passive-first active-last process flow showing how the IC fabrication can be integrated into standard Si BEOL process. Four metal levels (M1–M4) are required to complete the circuit. ( b ) Tilted view scanning electron microscopic (SEM) image revealing the integration of key components in IC with enlarged view showing the advanced gate structure of the graphene field-effect transistors (GFET). Inset image shows cross-sectional SEM of embedded T-shaped gate. Scale bar, 500 nm. Full size image To illustrate the integration architecture, a tilted view scanning electron microscopic image capturing key circuit components from the wafer completing the gate fabrication, before graphene transfer, is shown in Fig. 1b . All the inter-metal dielectrics as well as gate dielectric were stripped off to reveal the underlying structure. The unique embedded T-shaped gate structure in Fig. 1b , together with the multiple-finger design, provides very low gate resistance while maintaining a short channel length, leading to notably improved f MAX verified from stand-alone RF transistors built on the same chip ( Supplementary Fig. 3 ) [22] . The IC consists of 11 components including 3 GFETs, 4 inductors, 2 capacitors and 2 resistors ( Fig. 2a,b ). The circuit is designed as an RF receiver front-end comprising three stages. Each stage is connected to the next through capacitive coupling; thus, the gate bias ( V g ) of each stage can be individually adjusted to optimize circuit performance. The first two stages are designed as band-pass amplifiers, providing amplification and filtering of received RF signal. The third stage performs mixing with LO signal that down-converts the GHz RF signal to much lower intermediate frequency (IF) in the MHz range. Although the ambipolar nature of graphene enables several new circuit designs [12] , [23] , including subharmonic mixer operation [14] , these mixers require the Dirac point close to zero gate bias with highly symmetric electron and hole transfer curves for the best performance, and relatively high levels of LO power. In our design, a fundamental drain-pumped mixer is employed since it leads to better performance based on the characteristics of our graphene transistors (shown in Fig. 2d–g ), and results in low LO power requirements (<0 dBm). Inductor L4, connected at the drain of mixing FET, serves a double purpose: it resonates the drain capacitance of transistor T3 to provide a large LO voltage swing at the drain terminal, and it attenuates the LO signal leakage towards the IF port. The photo of a fabricated chip in Fig. 2c exhibits arrays of graphene ICs, transistors for S-parameter characterization and process monitor structures ( Supplementary Fig. 4 ). 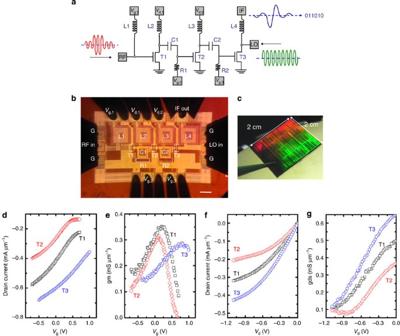Figure 2: Circuit diagram and device DC performance. (a) Circuit schematic of three-stage graphene receiver IC comprising 11 active and passive components. (b) Optical micrograph of an IC under testing. The circuit has the dimension of 1,020 × 600 μm2. Scale bar, 100 μm. (c) Photo of a fully processed graphene IC chip. (d) Drain currents as a function of gate biases for three transistors in one circuit and (e) their width normalized transconductances. The drain biases were −1 V. (f) Drain currents as a function of drain biases and (g) width normalized output conductances from the same devices. The gate biases were 0.25 V for both devices T1 and T2, and 0.75 V for device T3. Figure 2: Circuit diagram and device DC performance. ( a ) Circuit schematic of three-stage graphene receiver IC comprising 11 active and passive components. ( b ) Optical micrograph of an IC under testing. The circuit has the dimension of 1,020 × 600 μm 2 . Scale bar, 100 μm. ( c ) Photo of a fully processed graphene IC chip. ( d ) Drain currents as a function of gate biases for three transistors in one circuit and ( e ) their width normalized transconductances. The drain biases were −1 V. ( f ) Drain currents as a function of drain biases and ( g ) width normalized output conductances from the same devices. The gate biases were 0.25 V for both devices T1 and T2, and 0.75 V for device T3. Full size image One key feature of this process flow is to fabricate GFET as the last step, which prevents possible graphene damage during harsh BEOL processes (for example, chemical mechanical polishing and Cu electroplating). This advantage can be clearly seen from direct current performance of three GFETs of gate lengths of 900 nm and device widths of 12 μm in one circuit measured after the full circuit has been built, as shown in Fig. 2 , where Fig. 2d,e and Fig. 2f,g present transfer and output characteristics, respectively. At −1 V drain bias ( V d ), these devices exhibit peak transconductance (gm) larger than 0.3 mS μm −1 , on par with state-of-the-art GFETs with similar device dimensions and about 450% better than the device in the previous graphene IC report despite a higher V d (1.6 V) was used [16] . More importantly, the devices show clear drain current saturation (verified by low output conductance (gds) in Fig. 2g ), leading to high intrinsic gain (gm gds −1 ) of about 2–4.5. We would like to point out that the gapless band structure in graphene typically causes the weaker saturation of the drain current in GFET compared with other semiconductor devices with a bandgap [24] . We have previously shown that by employing a very thin gate dielectric (equivalent oxide thickness less than 2 nm), full drain current saturation (gds=0) can be achieved in GFETs [25] . Therefore, a higher gain performance can be expected by continuously improving the gate dielectric quality in our IC fabrication process. At 1 V drain bias, f T and f MAX ranging from 8 to 10 GHz and from 8.5 to 13.5 GHz, respectively, were measured from stand-alone RF transistors with the same gate length. It is noteworthy that the current chips have not gone through the last passivation step. Several reports have shown that various dielectric films can be directly deposited on graphene, such as Si 3 N 4 deposited by plasma-enhanced CVD [26] or a NO 2 and HfO 2 stack deposited by ALD [27] , which can provide sufficient chip protection. IC performance Before testing the IC as an RF receiver, the successful circuit integration was verified by measuring it as an RF amplifier driving a 50-Ω load, a standard impedance in RF systems. A small-signal power gain of 10 dB at 1 GHz has been previously demonstrated with a discrete graphene transistor [28] . This circuit function in our IC can be achieved by simply adjusting gate biases of transistors to their highest gm points, and replacing the IF output in Fig. 2a with the third-stage drain bias. 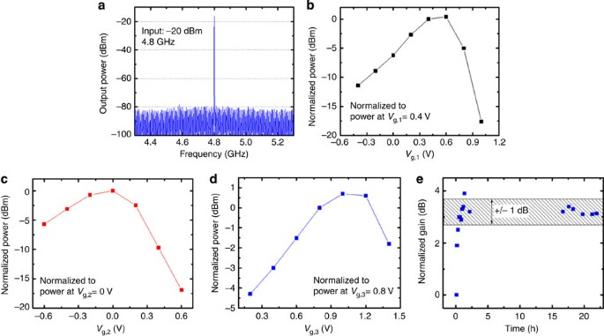Figure 3: Graphene IC measured as RF amplifier. (a) Output spectrum of the IC with 900 nm gate length under −1.6 VVdwith input power of −20 dBm at 4.8 GHz. (b) Normalized amplifier output power as a function of the first-stage gate bias (Vg,1). The second-stage gate bias (Vg,2) was kept at −0.13 V and the third-stage gate bias (Vg,3) was kept at 0.99 V. (c) Normalized amplifier output power as a function ofVg,2.Vg,1=0.45 V andVg,3=0.99 V. (d) Normalized amplifier output power as a function ofVg,3.Vg,1=0.45 V andVg,2=−0.13 V. (e) Variation of amplifier gain during bias stress test for over 22 h. The circuit was measured in air. Figure 3a shows that the IC exhibits +4 dB power gain, which is the first graphene IC able to perform amplification when loaded with 50 Ω impedance. This performance is in good agreement with circuit simulations performed using the measured values of individual components ( Supplementary Fig. 5 , Supplementary Note 1 ). To demonstrate that each of the three active stages is operational, Fig. 3b–d shows the normalized gain as a function of V g in one stage while keeping V g of other two stages constant. The gain of each stage can be independently controlled, confirming the correct functions from all active and passive components in each stage. In addition, the stability of the graphene IC was tested by applying high drain current stress and monitoring the gain variation continuously ( Fig. 3e ). The initial performance improvement is attributed to the current-induced annealing effect that removes contamination of graphene [29] . Once transistors become stabilized, the circuit exhibits less than ±1 dB variation during >20 h testing period, suggesting excellent stability and reliability. Figure 3: Graphene IC measured as RF amplifier. ( a ) Output spectrum of the IC with 900 nm gate length under −1.6 V V d with input power of −20 dBm at 4.8 GHz. ( b ) Normalized amplifier output power as a function of the first-stage gate bias ( V g,1 ). The second-stage gate bias ( V g,2 ) was kept at −0.13 V and the third-stage gate bias ( V g,3 ) was kept at 0.99 V. ( c ) Normalized amplifier output power as a function of V g,2 . V g,1 =0.45 V and V g,3 =0.99 V. ( d ) Normalized amplifier output power as a function of V g,3 . V g,1 =0.45 V and V g,2 =−0.13 V. ( e ) Variation of amplifier gain during bias stress test for over 22 h. The circuit was measured in air. Full size image The circuit was measured in receiver mode, with an LO signal applied at the drain of T3 and IF output measured after L4. The measured output spectrum is shown in Fig. 4a . The conversion gain of the circuit with 4.3 GHz RF input signal is −10 dB with a low LO input power ( P LO ) of −2 dBm, presenting 50 times higher conversion gain with 200 times smaller LO power compared with previously reported graphene IC ( Supplementary Table 2 ) [16] . Such low P LO is important to effectively prevent LO from leaking into the final IF output. The measured conversion gain as a function of P LO is also shown in Supplementary Fig. 6 . With drain biases of −1.5 V, the whole three-stage IC consumes less than 20 mW power, 600% lower than single-stage graphene IC in ref. 16 . 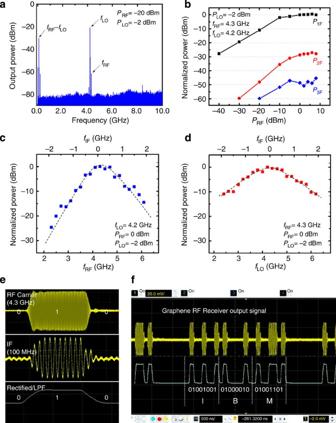Figure 4: Graphene IC measured as RF receiver. (a) Output spectrum of graphene receiver with 900 nm gate length. RF input signal was −20 dBm at 4.3 GHz and LO input signal was −2 dBm at 4.2 GHz. Down converted IF output signal at 100 MHz (fIF=fRF−fLO) was −30 dBm. (b) Normalized output power of the fundamental tone (P1F), the second harmonic (P2F) and the third harmonic (P3F) as a function of RF power (PRF), showing no gain compression up to −10 dBmPRF. (c) Normalized output power as a function of LO frequency. (d) Normalized output power as a function of RF. (e) Measured waveforms of RF input signal amplitude modulated at a rate of 20 Mb s−1, IF output signal and restored binary code after rectifying and low-pass filtering IF signal. (f) A screenshot of receiver output waveforms taken from the oscilloscope, with LO power of −2 dBm at 4.2 GHz. The original bit stream comprising three letters (24 bits) was recovered by graphene receiver with very low distortion. The circuit was measured in air. Figure 4b shows the measured receiver output tones ( P 1F , P 2F , P 3F ) as a function of input RF power ( P RF ); low RF harmonic distortion ( P 1F – P 2F ~30 dB for P RF =0 dBm) indicates good circuit linearity. The circuit is designed to band-pass filter the RF input signal before entering the mixer to improve the data quality by rejecting unwanted signals outside the carrier frequency band. The effective RF input filtering can be seen from the sharp frequency response in Fig. 4c (~1 GHz of 3-dB bandwidth). The receiver conversion gain is also measured as a function of the LO frequency ( Fig. 4d ). Figure 4: Graphene IC measured as RF receiver. ( a ) Output spectrum of graphene receiver with 900 nm gate length. RF input signal was −20 dBm at 4.3 GHz and LO input signal was −2 dBm at 4.2 GHz. Down converted IF output signal at 100 MHz ( f IF = f RF − f LO ) was −30 dBm. ( b ) Normalized output power of the fundamental tone ( P 1F ), the second harmonic ( P 2F ) and the third harmonic ( P 3F ) as a function of RF power ( P RF ), showing no gain compression up to −10 dBm P RF . ( c ) Normalized output power as a function of LO frequency. ( d ) Normalized output power as a function of RF. ( e ) Measured waveforms of RF input signal amplitude modulated at a rate of 20 Mb s −1 , IF output signal and restored binary code after rectifying and low-pass filtering IF signal. ( f ) A screenshot of receiver output waveforms taken from the oscilloscope, with LO power of −2 dBm at 4.2 GHz. The original bit stream comprising three letters (24 bits) was recovered by graphene receiver with very low distortion. The circuit was measured in air. Full size image To best demonstrate the true functionality of the graphene IC, an RF carrier of 4.3 GHz was amplitude modulated with a bit stream and sent into the receiver to mimic the typical digital data transmitted via wireless carrier. Measured single bit waveforms in Fig. 4e show undistorted IF output signal from the receiver without the aid of any additional signal amplification, suggesting that a high-quality receiver function has been achieved. The original binary code can then be easily recovered by rectification and low-pass filtering. Figure 4f further shows that bit stream comprising ASCII code of ‘IBM’ modulated at 20 Mb s −1 is successfully received and demodulated. The modulation rate is limited by the test equipment, and not by the receiver IC. The demonstration of multifunctional RF ICs built with the graphene-last flow in Si fab clearly paves the way for seamless heterogenous three-dimensional (3D) system integration, where graphene IC’s BEOL can be co-integrated with standard Si CMOS BEOL as illustrated in Fig. 1a . On the other hand, stacking conventional semiconductor layers such as Si or III-V into 3D system is rather complicated and costly, where challenges arise from high-temperature annealing processes (typically>1,000 °C) required for each active layer device formation that are not compatible to Cu BEOL technology [30] . Our entire IC fabrication flow does not require any process steps higher than 400 °C, making it an ideal candidate for monolithic 3D integration with Si CMOS backbone. Such integration concept fully utilizes the transfer property of graphene, and one can envision that high-performance graphene RF circuits will be directly built on top of high-density Si CMOS logic circuits to form an extremely low-cost, ultra-compact communication system. CVD graphene growth and transfer The graphene growth was carried out in a 4-inch furnace, which can support up to 12 × 12 inch 2 graphene size. A Cu foil (99.99% from Kamis) was annealed at 1,050 °C for 5 min in 5 mTorr CH4 for initial graphane island growth, and then annealed for 20 min in 75 mTorr CH4 for graphene growth [18] . The graphene was transferred to a target substrate with typical wet transfer process. First, 150 nm thick PMMA was spin coated on the graphene/Cu foil sample (3,000 r.p.m. for 1 min). The polymethyl methacrylate (PMMA)/graphene/Cu foil sample was then floated on 1 M FeCl3 to dissolve the Cu foil, followed by moving the remaining PMMA/graphene sample on 1 M HCl for rinsing away the residue of Cu etchant. Finally, the PMMA/graphene sample was scooped by a target substrate and then blown dry by pure nitrogen. Passive-first active-last process flow A total of nine lithography masks are required to complete the IC fabrication. In a 200-mm silicon fab, beginning with low-doped Si wafers with 2 μm thick silane oxide deposition at 400 °C, the wafer was then spin coated with photoresist and patterned using an ASML Deep ultraviolet stepper. High-power reactive ion etching (RIE) with a mixture of C 4 F 8 and Ar for 135 s was used to remove ≈1 μm SiO 2 , and the photoresist was stripped off in oxygen plasma. Physical vapour deposited liner consisting of TaN/Ta was adapted before the deposition of a thin Cu seed layer, which was followed by Cu electroplating and chemical mechanical polishing. After inspection of post-CMP patterns, low-stress CVD nitride (100 nm) and silane oxide (800 nm) were deposited. The measured capacitance of plate capacitors is 6.1 × 10 3 pF cm −2 . Cu vias and following metal levels were fabricated using similar process steps with different dielectric thickness and etch time. Al 2 O 3 gate dielectric (100 Å) was then deposited at 250 °C using TMA and H 2 O in a Fiji ALD system to cover the whole wafer and an HBr-based RIE process was used to etch open the contact pad to the gate. After CVD-grown graphene was transferred, photoresist was again patterned in a DUV system and the exposed graphene area was etched away in a Unaxis RIE system with a 50-W plasma maintained by 30 s.c.c.m. O 2 . Photolithographic patterning was used to define source/drain electrodes and electron beam evaporation was used to sequentially deposit 0.2 nm Ti, 20 nm Pd and 30 nm Au followed by a lift-off process in resist stripper. IC measurement The LO signal was provided by a Wiltron 69047A signal generator, and the input RF signal was provided by a Rohde & Schwarz SMIQ06B signal generator, which could be 100% amplitude modulated to about 20 MHz by an external signal. The mixer and amplifier outputs were measured with an Agilent E4448A spectrum analyser. Losses due to bias tees, cables and probe resistance were calibrated using an on-wafer ‘through’ wire structure. Modulation of the input RF signal was performed by driving the RF signal generator amplitude modulation input with a data pattern stored on an Agilent 81133 pulse generator. The demodulated signal was observed on an Agilent DSA91204A real-time oscilloscope, which also performed the rectification and low-pass filtering to convert it to digital format. How to cite this article: Han, S.-J. et al. Graphene radio frequency receiver integrated circuit. Nat. Commun. 5:3086 doi: 10.1038/ncomms4086 (2014).